Reducing the impact of intrinsic dissipation in a superconducting circuit by quantum error detection A fundamental challenge for quantum information processing is reducing the impact of environmentally induced errors. Here we demonstrate a quantum error detection and rejection protocol based on the idea of quantum uncollapsing, using this protocol to reduce the impact of energy relaxation owing to the environment in a three-qubit superconducting circuit. We encode quantum information in a target qubit, and use the other two qubits to detect and reject errors caused by energy relaxation. This protocol improves the storage time of a quantum state by a factor of roughly three, at the cost of a reduced probability of success. This constitutes the first experimental demonstration of the algorithm-based improvement in the lifetime of a quantum state stored in a qubit. Superconducting quantum circuits are very promising candidates for building a quantum processor owing to the combination of good qubit performance and the scalability of planar integrated circuits [1] , [2] , [3] , [4] , [5] , [6] , [7] , [8] , [9] , [10] . In addition to recent, very significant improvements in the materials and qubit geometries in such circuits, external control and measurement protocols are being developed to improve performance. This includes the use of dynamical decoupling [11] , measurement-based feedback controls [12] , [13] and preliminary experiments [14] with quantum error correction (QEC) codes, which allow the removal of artificially induced errors [14] , [15] , [16] , [17] , [18] . To date, however, there has been little experimental progress in control sequences that reduce a significant source of qubit error: energy dissipation due to the environment. Although there are QEC proposals to correct intrinsic dissipation errors [18] , [19] , these have not yet been demonstrated experimentally, mostly due to gate fidelity limitations. Quantum error detection and rejection (QEDR) [20] , [21] provide an alternative, albeit non-deterministic approach to handling errors, avoiding some of the complexity of full QEC by simply rejecting errors when they are detected. Using a variant of quantum uncollapsing that combines a weak measurement with its reversal [22] , [23] , [24] , [25] , QEDR has been predicted to significantly reduce the impact of energy relaxation in qubits [21] , one of the dominant sources of error in superconducting quantum circuits [1] , [2] , [3] . The QEDR protocol based on uncollapsing [22] is illustrated in Fig. 1a . Starting with a qubit in a superposition of its ground | g › and excited | e › states, | ψ i ›= α | g ›+ β | e ›, a weak measurement is performed that detects the | e › state with probability (measurement strength) p <1. In the null-measurement outcome (| e › state not detected), this produces the partially collapsed state | ψ 1 ›= α | g ›+ β | e › (the squared norm equals the outcome probability). The system is then stored for a time τ , during which it can decay (jump) to the | g › state or remain in the no-jump state | ψ nj ›= α | g ›+ β e − Γτ /2 | e ›, where Γ =1/ T 1 is the energy relaxation rate. (Instead of using the master equation formalism for the density matrix to account for the energy relaxation, here we prefer to use the Kraus operator-based jump and no-jump scenarios, as this gives more physical insight. See Supplementary Notes 2 and 3 , and elsewhere [21] , [22] for details.) The uncollapsing measurement is then performed, comprising a π x rotation and a second weak measurement with strength p u , followed by a final π x rotation that undoes the first rotation. Only outcomes that yield a second null measurement are kept. 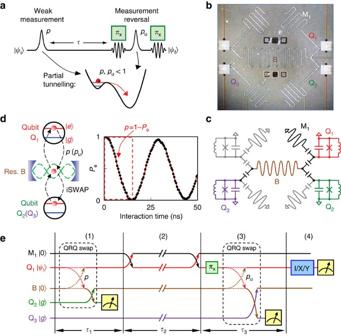Figure 1: Device geometry and uncollapsing protocol used for QEDR. (a) Quantum uncollapsing protocol in the phase qubit22,23. Top: pulse sequence, where the weak measurement with strengthpis followed by a delay (storage time)τ, and then the measurement reversal, involving aπxrotation, a weak measurement with strengthpu, and a secondπxrotation. Bottom: the delta-like electrical pulses lower the tunnel barrier for the qubit states on the left of the potential landscape to allow partial tunnelling of the |estate into the well on the right. (b,c) Optical micrograph and simplified schematic of the device. Circuit elements are as labelled; those not used in this experiment are in grey. (d) Illustration of the qubit–resonator–qubit (QRQ) swap, analogous to the partial tunnelling measurement. Left: schematic for the sequential qubitQ1-resonatorBswap with swap probability (measurement strength)p(pu), followed by a full iSWAP between resonatorBand qubitQ2(Q3). Right: the on-resonance, unit-amplitude qubit-resonator vacuum Rabi oscillations in the qubit |estate probabilityPe(vertical axis), starting with the qubit in |eand resonator in |0. The measurement strengthp=1−Peis set by the interaction time (horizontal axis). (e) QEDR protocol, where we start withQ1in |ψi, consisting of the following steps: (1) the first weak measurement is performed using the first QRQ swap involvingQ1–B–Q2, with strengthp.Q2is measured immediately, and only null outcomes (Q2in |g) are accepted. (2) The state is swapped fromQ1into memory resonatorM1and stored for a relatively long timeτ2, following which the state is swapped back intoQ1. (3) The weak measurement reversal is performed using aπxrotation onQ1and a second QRQ swap with strengthputo qubitQ3.Q3is then measured, and only null outcomes (Q3in |g) are accepted. (4) The double-null outcomes are analysed using tomography ofQ1to evaluateQ1’s final density matrix. To save time and reduce errors, we do not perform the finalπxrotation appearing in the full uncollapsing protocol. These double-null outcomes give the result | ›=| g › if the system jumped to | g › during the time interval τ , while in the no-jump case, the final state is Figure 1: Device geometry and uncollapsing protocol used for QEDR. ( a ) Quantum uncollapsing protocol in the phase qubit [22] , [23] . Top: pulse sequence, where the weak measurement with strength p is followed by a delay (storage time) τ , and then the measurement reversal, involving a π x rotation, a weak measurement with strength p u , and a second π x rotation. Bottom: the delta-like electrical pulses lower the tunnel barrier for the qubit states on the left of the potential landscape to allow partial tunnelling of the | e state into the well on the right. ( b , c ) Optical micrograph and simplified schematic of the device. Circuit elements are as labelled; those not used in this experiment are in grey. ( d ) Illustration of the qubit–resonator–qubit (QRQ) swap, analogous to the partial tunnelling measurement. Left: schematic for the sequential qubit Q 1 -resonator B swap with swap probability (measurement strength) p ( p u ), followed by a full iSWAP between resonator B and qubit Q 2 ( Q 3 ). Right: the on-resonance, unit-amplitude qubit-resonator vacuum Rabi oscillations in the qubit | e state probability P e (vertical axis), starting with the qubit in | e and resonator in |0 . The measurement strength p =1− P e is set by the interaction time (horizontal axis). ( e ) QEDR protocol, where we start with Q 1 in | ψ i , consisting of the following steps: (1) the first weak measurement is performed using the first QRQ swap involving Q 1 – B – Q 2 , with strength p . Q 2 is measured immediately, and only null outcomes ( Q 2 in |g ) are accepted. (2) The state is swapped from Q 1 into memory resonator M 1 and stored for a relatively long time τ 2 , following which the state is swapped back into Q 1 . (3) The weak measurement reversal is performed using a π x rotation on Q 1 and a second QRQ swap with strength p u to qubit Q 3 . Q 3 is then measured, and only null outcomes ( Q 3 in |g ) are accepted. (4) The double-null outcomes are analysed using tomography of Q 1 to evaluate Q 1 ’s final density matrix. To save time and reduce errors, we do not perform the final π x rotation appearing in the full uncollapsing protocol. Full size image Remarkably, the final no-jump state is identical to | ψ i › if we choose 1− p u =(1− p ) e − Γτ ; the probability of this (desired) outcome is =‹ | ›=(1− p ) e − Γτ , while the probability of the undesirable jump outcome | g › is =| β | 2 (1− p ) 2 e − Γτ (1− e − Γτ ). These two probabilities do not add to one; the remaining probability covers situations other than these double-null measurement outcomes. As the probability P f j falls to zero more quickly than as p →1, increasing the measurement strength p towards 1 results in a higher likelihood of recovering the initial state. This comes at the expense of a low probability P DN = + of the double-null result. The resulting density matrix is ρ f =( | ›‹ |+ | g ›‹ g |)/ P DN . The QEDR protocol in Fig. 1a relies on partial tunnelling to perform the weak measurement. We have performed the protocol in this way, but found that this gave low fidelities. We therefore, in addition, implemented a weak measurement using a partial swap between the target qubit and an ancilla qubit, followed by a projective measurement of the ancilla; the two weak measurements in the QEDR protocol thus required two ancilla qubits. Using this alternative measurement, here we show that a quantum state suffering from dissipation errors can be almost fully recovered, although only by rejecting a large fraction of the measurement outcomes. This allowed us to extend the intrinsic lifetime of a quantum state by a factor of about three. A somewhat similar protocol has been demonstrated with photonic qubits, but only to suppress intentionally generated errors [26] . Implementation of the weak measurement The device we used to implement the QEDR protocol is similar to that in Lucero et al. [27] (shown in Fig. 1b,c ), with three phase qubits, Q 1 , Q 2 and Q 3 , coupled to a common, half-wavelength coplanar waveguide bus resonator B , with a memory resonator M 1 also coupled to Q 1 . Relevant parameters are tabulated in Supplementary Table 1 (see Supplementary Note 1 for sample fabrication details). The partial measurement method is illustrated in Fig. 1d . Qubit Q 1 is the target, and Q 2 and Q 3 are ancillae, entangled with Q 1 via the resonator bus B , such that a projective measurement of Q 2 or Q 3 results in a weak measurement of Q 1 . The entanglement begins with a partial swap between Q 1 and the resonator B : When qubit Q 1 , initially in | e ›, is tuned to resonator B , the probability P e of finding the qubit in | e › oscillates with unit amplitude at the vacuum Rabi frequency [28] , [29] , [30] . A partial swap with swap probability p =1− P e is achieved by controlling the interaction time, entangling Q 1 and B . We then use a complete swap (an iSWAP) between resonator B and qubit Q 2 ( Q 3 ), transferring the entanglement, followed by a projective measurement of Q 2 ( Q 3 ). In general, we start with Q 1 in | ψ i ›= α | g ›+ β | e › and perform the qubit–resonator–qubit (QRQ) swap, followed by measurement of the ancilla. A null outcome ( Q 2 or Q 3 in | g ›) yields the Q 1 state α | g ›+ β | e ›, as with partial tunnelling. The swap probability p is therefore equivalent to the measurement strength. Full QEDR sequence Our QEDR protocol can protect against energy decay of the quantum state. However, as dephasing in these qubits is an important error source, against which the QEDR protocol does not protect, we store the intermediate quantum state in the memory resonator M 1 , which does not suffer from dephasing (as indicated by T 2 ≅ 2 T 1 for the resonator; see Supplementary Table 1 ). Our full QEDR protocol is thus shown in Fig. 1e , starting with the initial state of the system as where | q 1 q 2 q 3 › represents the state of the qubits Q 1 , Q 2 and Q 3 , with the ground state |00› of the B and M 1 resonators listed last. In step 1, we use a QRQ swap between Q 1 , B and Q 2 with swap probability (measurement strength) p , followed immediately by measurement of Q 2 . This step takes a time τ 1 of up to 15 ns, depending on p . A null outcome ( Q 2 in | g ›) yields |ψ 1 ›= α | ggg ›|00›+ β | egg ›|00› (a more precise expression appears in Supplementary Note 2 ). In step 2, we swap the quantum state from Q 1 into M 1 , wait a relatively long time τ = τ 2 , during which the state in M 1 decays at a rate Γ =1/ T 1 , and we then swap the state back to Q 1 . In the no-jump case, the state becomes | ›= α | ggg ›|00›+ β | egg ›|00›. We then perform step 3, comprising a π x rotation on Q 1 followed by the second QRQ swap with strength p u , involving Q 1 , B and Q 3 , which takes a time τ 3 . τ 3 is between 20 and 35 ns, depending on p u , dominated by the 20 ns-duration π x pulse. Q 3 is then measured, with a null outcome ( Q 3 in | g ›) corresponding to We recover the initial state |ψ i › if we set 1− p u =(1− p ) e − Γτ 2 , with the undesired jump cases mostly eliminated by the double-null selection. To shorten the sequence, we do not perform the final π x rotation, so the amplitudes of Q 1 ’s | g › and | e › states are reversed compared with the initial state. In step 4, we apply tomography pulses and then measure Q 1 to determine its final state, keeping the results that correspond to the double-null outcomes ( Q 2 and Q 3 in | g ›). Characterizing the QEDR performance We use quantum process tomography to characterize the performance of the protocol, starting with the four initial states {| g ›, | g ›− i | e ›, | g ›+| e ›, | e ›} and measuring the one-qubit process matrix χ . As we reject outcomes, where Q 2 and Q 3 are not measured in | g ›, the process is not trace preserving, so the linear map satisfies ρ f P DN = , where ρ i and ρ f are the normalized initial and final density matrices of Q 1 , and E n is the standard Pauli basis {I,X,Y,Z}. We define the process fidelity as [31] =Tr( χ ideal χ )/Tr( χ ), where χ ideal corresponds to the desired unitary operation (here given by π x ), and the divisor accounts for postselection. There are other ways to define the process fidelity F ; for instance, one can average the state fidelity over a set of pure initial states, either with or without weighting by the selection probability [21] , [32] . We have analysed the data using various definitions of the fidelity and found similar fidelity improvement due to QEDR for all of them. See Supplementary Note 4 for more details. We first tested the process with no storage, entirely omitting step 2 in Fig. 1e , and choosing p u = p ; we also delayed the measurement of Q 2 to the end of step 3 to minimize crosstalk (see Methods). 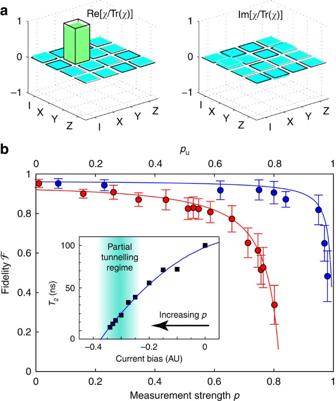Figure 2: Fidelity of the uncollapsing protocol without storage. (a) Measuredχ/Tr(χ) (bars with colour), whereχis the non-trace-preserving quantum process tomography matrix for the sequence inFig. 1eexcluding step 2, here withp=pu=0.75. The desired matrix,χideal, corresponds to aπrotation about the Bloch spherexaxis (identified by black frames). (b) Process fidelity for both the three-qubit QRQ-based uncollapsing (blue circles) and the single-qubit partial-tunnelling version (red circles)23, both as a function ofp=pu. Statistical errors are shown by error bars, defined as ±1 s.d., using the repeated sets of fidelity measurement. The process fidelity is above 0.9 forp≤0.8 using the QRQ swaps, while for the partial-tunnelling scheme it decreases significantly forp≥0.5. This decrease is primarily due to reduction in qubitT2with measurement current bias, shown in the inset; partial tunnelling occurs in the shaded region. Blue line is a simulation usingκ1=κ3=0.985,κ2=1, andκϕ=0.95 (seeSupplementary Note 3); the red line is a guide to the eye. Figure 2a shows the measured χ /Tr( χ ) for p = p u =0.75; the calculated process fidelity is =0.92. In Fig. 2b , we show the measured process fidelity as a function of the QRQ measurement strength p = p u (blue circles). Figure 2: Fidelity of the uncollapsing protocol without storage. ( a ) Measured χ /Tr( χ ) (bars with colour), where χ is the non-trace-preserving quantum process tomography matrix for the sequence in Fig. 1e excluding step 2, here with p = p u =0.75. The desired matrix, χ ideal , corresponds to a π rotation about the Bloch sphere x axis (identified by black frames). ( b ) Process fidelity for both the three-qubit QRQ-based uncollapsing (blue circles) and the single-qubit partial-tunnelling version (red circles) [23] , both as a function of p = p u . Statistical errors are shown by error bars, defined as ±1 s.d., using the repeated sets of fidelity measurement. The process fidelity is above 0.9 for p ≤0.8 using the QRQ swaps, while for the partial-tunnelling scheme it decreases significantly for p ≥0.5. This decrease is primarily due to reduction in qubit T 2 with measurement current bias, shown in the inset; partial tunnelling occurs in the shaded region. Blue line is a simulation using κ 1 = κ 3 =0.985, κ 2 =1, and κ ϕ =0.95 (see Supplementary Note 3 ); the red line is a guide to the eye. Full size image We can compare our no-storage uncollapsing fidelity to that obtained using partial tunnelling for the weak measurement of a single qubit [23] , shown in Fig. 2b (red circles). We see that even though the QRQ-based protocol is more complex, it achieves much better fidelities for p ≥0.5. This is mostly because of strong dephasing and two-level state effects [4] , [29] during the partial tunnelling current pulse (see inset in Fig. 2b ). Protection from energy relaxation We then tested the full QRQ protocol’s ability to protect from energy decay. The uncollapsing strength p u is given by [22] 1− p u =(1− p ) κ 1 κ 2 / κ 3 , where κ 2 =exp(− τ 2 / T 1 ), and κ 1 and κ 3 are similar energy relaxation factors for the steps 1 and 3 (here κ 1 ≈ κ 3 ≈0.985; see Supplementary Note 3 ). In Fig. 3a , we display the measured fidelities for the storage durations τ 2 =0.9, 1.7 and 3 μs for the memory resonator with T 1 =2.5 μs, compared with simulations using the pure dephasing factor κ ϕ =0.95 (see Korotkov and Keane [22] and Supplementary Note 3 ). The simulations are in excellent agreement with the data, and we see a marked improvement in the storage fidelity using QEDR over that of free decay (dashed line in each panel). 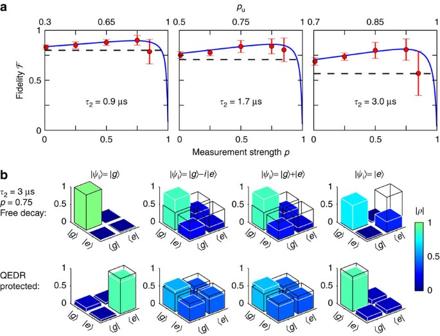Figure 3: QEDR-based quantum state protection from energy relaxation. (a) Process fidelity as a function of measurement strengthpfor the full QEDR protocol for three storage timesτ2=0.9, 1.7 and 3 μs in a memory resonatorM1(T1=2.5 μs). The uncollapsing swap probabilitypuis indicated on the top axis (see text). Circles with error bars are measured data; lines are simulations (seeSupplementary Note 3). Horizontal dashed lines in each panel give the free-decay process fidelity; the improvement from QEDR is most significant for largerτ2. Error bars represent statistical errors (s.d.). These statistical errors increase with increasing QRQ measurement strengthp, mainly due to the decrease in sample size (fewer double-null outcomes), while errors due to uncertainties inpuare less than 10% of those shown in the figure (seeSupplementary Note 3); we compensate for dynamic phases (seeSupplementary Note 3). (b) Final density matrices (bars with colour) without (top row) and with (bottom row) QEDR, withp=0.75, for the four initial states as labelled, following aτ2=3 μs storage time (=0.3). The desired error-free density matrices are shown by black frames. We only display the absolute values of the density matrix elements |ρ|. Note that the QEDR-protected final states differ from the initial state by aπrotation. Figure 3: QEDR-based quantum state protection from energy relaxation. ( a ) Process fidelity as a function of measurement strength p for the full QEDR protocol for three storage times τ 2 =0.9, 1.7 and 3 μs in a memory resonator M 1 ( T 1 =2.5 μs). The uncollapsing swap probability p u is indicated on the top axis (see text). Circles with error bars are measured data; lines are simulations (see Supplementary Note 3 ). Horizontal dashed lines in each panel give the free-decay process fidelity; the improvement from QEDR is most significant for larger τ 2 . Error bars represent statistical errors (s.d.). These statistical errors increase with increasing QRQ measurement strength p , mainly due to the decrease in sample size (fewer double-null outcomes), while errors due to uncertainties in p u are less than 10% of those shown in the figure (see Supplementary Note 3 ); we compensate for dynamic phases (see Supplementary Note 3 ). ( b ) Final density matrices (bars with colour) without (top row) and with (bottom row) QEDR, with p =0.75, for the four initial states as labelled, following a τ 2 =3 μs storage time ( =0.3). The desired error-free density matrices are shown by black frames. We only display the absolute values of the density matrix elements | ρ |. Note that the QEDR-protected final states differ from the initial state by a π rotation. Full size image It is interesting to note that in Fig. 3a , the process fidelity is significantly improved even for zero measurement strength p =0 (note that p u >0), implying that a simpler QEDR protocol still provides some protection against energy relaxation. Another way to test QEDR is to monitor the evolution of individual quantum states. In Fig. 3b , we display the final density matrices measured either without (top row) or with (bottom row) QEDR, for four initial states in Q 1 , with storage in the memory M 1 for τ 2 ≈3 μs. Other than for the initial ground state | g ›, which does not decay, we see that the QEDR-protected states are much closer to the desired outcomes than the free-decay states (note the π rotation). If we look at the off-diagonal terms in the middle panels, they have decayed from 0.5 to about 0.4; this decay takes about 1.1 μs without QEDR, so the lifetime is increased by 3 μs/1.1 μs≈3. Also, if we look at Fig. 3a , the free-decay fidelity at 0.9 μs (left panel) is about the same as the maximum QEDR fidelity at 3.0 μs (right panel), also giving a factor of three improvement. The price paid for the lifetime improvement is the small fraction of outcomes accepted by the QEDR postselection, shown in Fig. 4 . The double-null probability P DN decreases with increasing measurement strength p for all initial states. A balance must therefore be struck between a larger T 1 improvement, occurring for larger p , and a larger fraction of accepted outcomes, which occurs for smaller p . 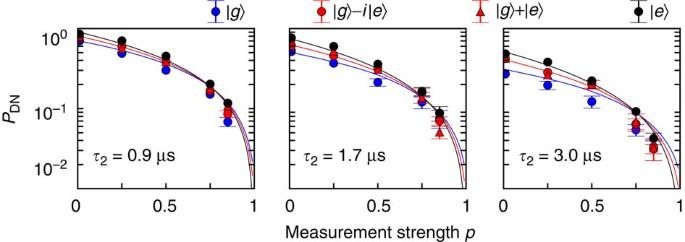Figure 4: QEDR selection probability. The QEDR protocol uses postselection to reject state decay errors. The probability of accepting an outcome, that is, the double-null probabilityPDN, falls with measurement strengthp. Here we displayPDNas a function ofp, corresponding to the data inFig. 3a, for each value of storage timeτ2. Error bars represent s.d. of repeated measurement results; error bars that are smaller than the symbol size are omitted for clarity. Lines are predicted by theory. Figure 4: QEDR selection probability. The QEDR protocol uses postselection to reject state decay errors. The probability of accepting an outcome, that is, the double-null probability P DN , falls with measurement strength p . Here we display P DN as a function of p , corresponding to the data in Fig. 3a , for each value of storage time τ 2 . Error bars represent s.d. of repeated measurement results; error bars that are smaller than the symbol size are omitted for clarity. Lines are predicted by theory. Full size image QEDR will be challenging to implement in large-scale qubit circuits, as it does not scale well, in particular when the fraction of successful outcomes is small; QEC, when it becomes an experimental reality, will clearly provide a far more efficient route to fault-tolerance, even though it requires significantly more resources (qubits and gates) than does QEDR (see Supplementary Note 5 ). However, the simplest QEC proposal for energy relaxation [19] is expected to only yield a factor of about two improvement in the state lifetime (assuming gate execution is almost perfect), which is less than the factor of three improvement demonstrated here using QEDR. The simpler QEDR protocol can therefore serve as a suitable intermediate to QEC, applicable to small and medium scale quantum circuits. Readout correction and crosstalk cancellation All data are corrected for the qubit readout fidelities before further processing. The readout fidelities for | g › ( F g ) and | e › ( F e ) of Q 1 , Q 2 and Q 3 are F 1g =0.95, F 1e =0.89, F 2g =0.94, F 2e =0.88, F 3g =0.94, F 3e =0.91, respectively. Crosstalk is another concern when performing QEDR to protect quantum states. We read out Q 2 immediately after the first QRQ swap in step 1 in Fig. 1e to avoid decay in Q 2 . However, due to measurement crosstalk in the qubit circuit, this measurement can result in excitations in resonator B ; while this does not directly affect the other qubits, we must reset the resonator prior to the second QRQ swap. This is done during the storage in the memory resonator by performing a swap between B and Q 3 , and then using a spurious two-level defect coupled to Q 3 to erase the excitation in Q 3 . As the storage time in M 1 is several microseconds, there is sufficient time to reset both B and Q 3 prior to the second QRQ swap. The intermediate reset of B could not be performed when doing the experiments in Fig. 2 , for which there is no storage interval. To avoid crosstalk in those measurements, we postponed the measurement of Q 2 until the end of the second QRQ sequence to step 3 of Fig. 1e . The | e › state probability in Q 2 drops by about 6% during this delay time, as estimated from Q 2 ’s T 1 . We have corrected for this drop when evaluating the Q 2 measurements for Fig. 2 . How to cite this article: Zhong, Y. P. et al. Reducing the impact of intrinsic dissipation in a superconducting circuit by quantum error detection. Nat. Commun. 5:3135 doi: 10.1038/ncomms4135 (2014).